Ambidextrous binding of cell and membrane bilayers by soluble matrix metalloproteinase-12 Matrix metalloproteinases (MMPs) regulate tissue remodelling, inflammation and disease progression. Some soluble MMPs are inexplicably active near cell surfaces. Here we demonstrate the binding of MMP-12 directly to bilayers and cellular membranes using paramagnetic NMR and fluorescence. Opposing sides of the catalytic domain engage spin-labelled membrane mimics. Loops project from the β-sheet interface to contact the phospholipid bilayer with basic and hydrophobic residues. The distal membrane interface comprises loops on the other side of the catalytic cleft. Both interfaces mediate MMP-12 association with vesicles and cell membranes. MMP-12 binds plasma membranes and is internalized to hydrophobic perinuclear features, the nuclear membrane and inside the nucleus within minutes. While binding of TIMP-2 to MMP-12 hinders membrane interactions beside the active site, TIMP-2-inhibited MMP-12 binds vesicles and cells, suggesting compensatory rotation of its membrane approaches. MMP-12 association with diverse cell membranes may target its activities to modulate innate immune responses and inflammation. Macrophages use macrophage elastase (matrix metalloproteinase-12; MMP-12) to overcome bacterial infections [1] , regulate antiviral immunity [2] and resolve inflammation [3] . The therapeutic potential of MMP-12 stems from its roles in smoking-induced emphysema [4] , abdominal aortic aneurysms [5] , atherosclerotic plaques [6] and viral infections [2] . More generally, MMPs modulate inflammation [3] , [7] , wound healing [8] , tumour microenvironments [9] , arthritis [10] , cardiovascular disease [11] , brain injury and synaptic remodelling [12] . Hence, the understanding of MMP mechanisms of action is critical for the development of targeted interventions. Among the 23 human MMPs, MMP-12 is one of the best understood and illustrates the conundrum of the compartmentalization of several of the water-soluble enzymes [12] , [13] . After MMP-12 is secreted by macrophages, it diffuses through extracellular spaces, where the protease can be inhibited, en route to virus-infected cells [2] . Yet MMP-12 activity was not observed in the aqueous milieu around activated macrophages, but rather near the cells’ surface [14] . Pericellular activity is consistent with MMP-12 shedding of tumour necrosis factor-α (TNF-α) from leukocytes in lungs exposed to smoke [15] . Remarkably, MMP-12 enters virus-infected cells and nuclei where it activates transcription to respond to viral infection [2] . Proteolysis by soluble MMP-8 and -9 occurs on neutrophil surfaces and surprisingly resists inhibition by tissue inhibitors of metalloproteinases (TIMPs) [16] , [17] . Purified plasma membranes harbour MMP-8 (ref. 17 ). MMP-7 binds epithelial and cancer cell surfaces and remains proteolytically active even with TIMPs present [18] . The findings that these soluble MMPs are active near cells, even when high-affinity TIMP inhibitors are present, range from being partly understood in the case of MMP-7 to completely mysterious in the case of MMP-12. Diverse mechanisms may recruit metalloproteinases to cell surfaces. MMP-7 is anchored to cells by heparan sulfate proteoglycans (CD44) and the cholesterol sulfate component of lipid rafts [18] , [19] , [20] , as well as binding vesicles [21] . Some soluble MMPs bind transmembrane proteins including αvβ3 and α2β1 integrins, tetraspanin CD151, CD44 and low-density lipoprotein receptor-related protein [13] , implying many means of localization. We set out to discover whether the well-characterized MMP-12 (refs 22 , 23 , 24 , 25 , 26 ) binds directly to lipid bilayers and plasma membranes of living cells. Our results take on unexpected relevance to the recent question of how active MMPs enter and move through cells [2] , [27] , [28] . To provide mechanistic insights, spin-labelled phospholipids in micelles were used to probe interactions with peripheral membrane proteins via paramagnetic NMR relaxation enhancements (PREs) [29] . Such PREs provide distance estimates that are useful for calculating realistic structures of the complexes. Disk-like, isotropic bicelles (bilayered micelles) are well-characterized [30] and offer a central bilayer and relatively fast tumbling for resolving NMR peaks. These membrane models yielded quantitative results with a peripheral membrane protein [31] and an integral membrane protein [32] , and are employed here. A polarity-sensitive fluorophore for detecting membrane interactions [33] , [34] and live cell imaging are applied as well. These strategies are integrated here to generate validated structures of complexes, revealing that MMP-12 consistently interacts in an ‘ambidextrous’ manner with bicelles, vesicles and various cellular membranes, using two non-contiguous surfaces. The unprecedented pair of membrane-binding surfaces position the active site and substrate access nearby, providing explanations for its pericellular proteolytic activities [14] , [15] , and potentially for the trafficking of this protease towards perinuclear and intranuclear compartments to shape innate immune and inflammatory responses [2] . Discovery of membrane-binding sites and complexes of MMP-12 To predict potential novel membrane-binding sites, we applied an experimentally trained algorithm called ‘membrane optimal docking area’ (MODA), which is now freely available at moda.ucsd.edu [35] , [36] . Application to the crystal structure of MMP-12 (PDB ID 1jk3) [37] predicted direct membrane binding by Gly167 to His172 of the III–IV loop and Gly188 to Gly192 of the IV–V loop due to the exposure of bilayer-interactive groups, particularly of Phe171 and Ile191 ( Fig. 1a ). 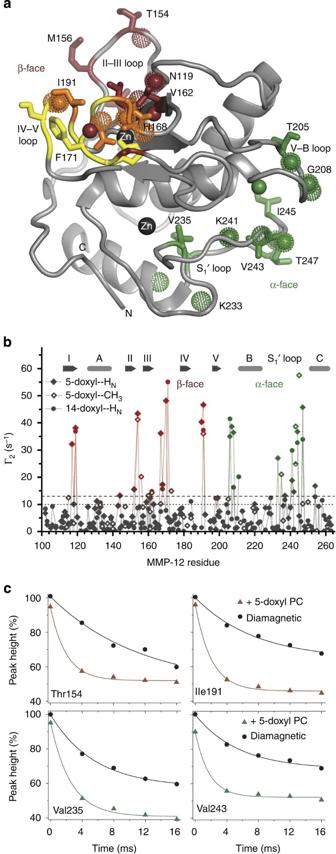Figure 1: MMP-12 associates with bilayer-mimicking bicelles via two distinct interfaces. (a) The MODA tool predicts membrane association with the residues of the IV–V and S-shaped III–IV loops, which are marked with yellow or orange ribbon and side chains. The proximities of MMP-12 groups to bicelles were measured using isotropic bicelles doped with nitroxide spin-labelled PC. This induces large NMR peak broadenings (PREs) to residues in two clusters highlighted in dark red/orange or green, respectively, on the NMR structure23. The 5-doxyl PC broadens the NMR line widths of amide protons marked with dots where Γ2>14 s−1and methyl groups with side chains plotted where Γ2>10 s−1. The more deeply buried spin label of 14-doxyl PC broadens the lines of amide protons plotted with spheres where Γ2>14 s−1. Orange marks residues with both PRE evidence and MODA prediction of bilayer interactions. Black spheres indicate zinc ions. (b) Close approaches of the protease to the bicelles are observed as PREs induced in amide and methyl protons by addition of nitroxide spin-labelled PC to one per leaflet of the isotropic bicelles. The PREs are plotted as Γ2relaxation rates. The colours correspond to the regions encompassing the two clusters indicated ina, with red representing the β-face and green the α-face. (c) Examples of methyl proton relaxation at the β-interface (upper panels) and α-interface (lower panels) with the membrane mimics are plotted with black circles for the diamagnetic control without addition or using coloured triangles with the addition of paramagnetic 5-doxyl PC. Figure 1: MMP-12 associates with bilayer-mimicking bicelles via two distinct interfaces. ( a ) The MODA tool predicts membrane association with the residues of the IV–V and S-shaped III–IV loops, which are marked with yellow or orange ribbon and side chains. The proximities of MMP-12 groups to bicelles were measured using isotropic bicelles doped with nitroxide spin-labelled PC. This induces large NMR peak broadenings (PREs) to residues in two clusters highlighted in dark red/orange or green, respectively, on the NMR structure [23] . The 5-doxyl PC broadens the NMR line widths of amide protons marked with dots where Γ 2 >14 s −1 and methyl groups with side chains plotted where Γ 2 >10 s −1 . The more deeply buried spin label of 14-doxyl PC broadens the lines of amide protons plotted with spheres where Γ 2 >14 s −1 . Orange marks residues with both PRE evidence and MODA prediction of bilayer interactions. Black spheres indicate zinc ions. ( b ) Close approaches of the protease to the bicelles are observed as PREs induced in amide and methyl protons by addition of nitroxide spin-labelled PC to one per leaflet of the isotropic bicelles. The PREs are plotted as Γ 2 relaxation rates. The colours correspond to the regions encompassing the two clusters indicated in a , with red representing the β-face and green the α-face. ( c ) Examples of methyl proton relaxation at the β-interface (upper panels) and α-interface (lower panels) with the membrane mimics are plotted with black circles for the diamagnetic control without addition or using coloured triangles with the addition of paramagnetic 5-doxyl PC. Full size image We tested these hypothetical sites using the catalytic domain, expressed without the prodomain and containing a stabilizing E219A mutation (‘MMP-12’), to represent the physiological state formed by rapid autolytic removal of the carboxyl-terminal (C-terminal) domain [38] . The proximity of MMP-12 residues to bicelles that mimic phospholipid membranes was measured by paramagnetic NMR. The isotope-labelled protease was introduced to bicelles containing phosphatidylcholine (PC) with dimyristoyl and dihexanoyl chains. Relaxation of amide and methyl NMR signals of MMP-12 was compared without and with addition of nitroxide spin-labelled PC to the bicelles mixed with the enzyme. The PC with either shallow 5-doxyl or deep 14-doxyl probe selectively broadens NMR peaks of Ala167, His168, Asp170, Phe171 and Ala173 with PREs, indicating that part of the III–IV loop to interact directly with bicelles ( Fig. 1 ). Likewise, the PREs of Gly190 and Ile191 indicate that the IV–V loop binds bicelles, again confirming the prediction. Accompanying bicelle-induced chemical shift perturbations further confirm these binding sites ( Supplementary Fig. 1a ). Neighbouring II–III loop residues Leu152, Thr154 and Met156 as well as Arg117 and Asn119 at the end of β-strand I also experience PREs from spin-labelled lipids in the bicelles ( Fig. 1 ). On the opposite side of the catalytic domain, the V–B loop at His206 to Gly208 and Asn211 and the S 1 ′ loop at Lys233, Val235, Lys241 to Asp244 and Thr247 also exhibit PREs. Surprisingly, this suggests two non-overlapping sites that can both bind bilayers, with one involving four loops around the β-sheet and the other comprising two loops on the opposite side of the active site cleft. The proximity of the bicelle-binding surfaces to either flank of the active site ( Fig. 1a ) and the proposed occlusion of MMP-7 and -26 active sites by non-physiological cationic liposomes [21] or detergent micelles [39] , respectively, raised the question of membrane occlusion of the MMP-12 active site. However, small unilamellar vesicles (SUVs) of zwitterionic 1,2-dimyristoyl- sn -glycero-3-phosphocholine (DMPC) that bind MMP-12 did not alter its peptidase activity ( Supplementary Fig. 1b ), indicating that the active site remains intact and accessible to peptide substrates. The open active site separated the PREs into two functionally significant sets, designated the β-interface for proximity to the β-sheet or the α-interface nearer the α-helices. The larger β-interface comprises of Thr115, Arg117, Asn119, Thr154, Met156, Leu160, Val162, Ala167, His168, Asp170, Phe171, Ala173, Gly190 and Ile191 ( Fig. 1 ). The α-interface includes Thr205 to Gly208, Asn211, Lys233, Val235, Lys241 to Ile245, Thr247, Leu250 and Asp254. Addition of the spin-labelled PC induced rapid relaxation of only around half of the NMR signal at either interface ( Fig. 1c ). This suggested that nearly equal populations of enzyme bound by way of the α- and β-interfaces to bicelles, that is, around half in each orientation. Due to the intrinsic uncertainties in the locations visited by a spin-labelled PC probe in a bicelle, the PRE-based distances were ambiguously restrained to eight alternative DMPC molecules within a bilayer model available [40] . Each significant PRE demonstrated proximity of that chemical group to the bicelle ( Fig. 1b ) and was converted using equation (1) into a group of distance restraints to the depth in both acyl chains in the eight DMPC molecules corresponding to the position of the nitroxide spin label. The structural calculations sought to satisfy any single restraint among each 16-member group of ambiguous depth restraints. Rigid-body docking of the β-face of the MMP-12 solution structure [23] to DMPC bilayer coordinates employed 352 ambiguous distance restraints between them, while the docking to the α-face used a non-overlapping set of 384 ambiguous restraints. These resulted in the distinct and well-converged starting structures of the complexes with DMPC bilayers that were refined by molecular dynamics (MD). Both orientations of MMP-12 stably converged on the fluid model bilayer ( Supplementary Movies 1 and 2 ). Ensembles of 14 representative structures were selected for best agreement with the PRE-derived depth restraints ( Fig. 2a,b ) with minimal violations ( Table 1 ). The backbone root mean squared deviation values to the mean structures of the β and α ensembles average 0.49 and 0.42 Å, respectively. The two structural ensembles differ in their orientations on the bilayer by 137°, and thus bind membranes via opposite sides of the enzyme. 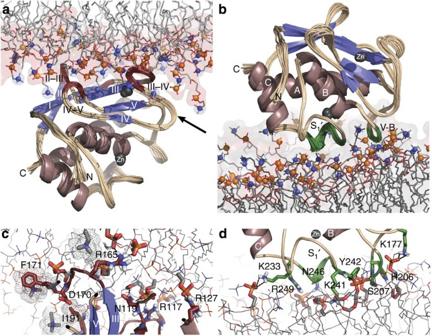Figure 2: PRE-NMR structural ensembles and interfacial contacts of DMPC bilayer bound to opposite sides of catalytic domain. (a) The ensemble of 14 structures of MMP-12 positioned with its β-face on the bilayer was selected from the MD trajectory ofSupplementary Movie 1. Backbone segments that contact the bicelles are coloured dark red. The view is illustrated as a stereo pair inSupplementary Fig. 9a. (b) The ensemble of 14 structures of MMP-12 bound with its α-face engaging the bilayer with green segments of the S1′ and V–B loops was selected from the MD trajectory ofSupplementary Movie 2. This view is illustrated as a stereo pair inSupplementary Fig. 9b. (c) A structure froma(viewed along the arrow ina) is marked with interfacial contacts which are populated in at least 64% of the final structures. Hydrophobic contacts are plotted with dot surfaces. Hydrogen bonds and salt bridges are plotted with broken lines. Nitrogen, phosphorous and oxygen atoms are coloured blue, gold and red, respectively. SeeSupplementary Fig. 2for a three-dimensional (3D), rotatable view. (d) A structure frombin the α orientation is marked with interfacial contacts reproduced in at least 64% of the final structures. SeeSupplementary Fig. 3for a 3D, rotatable view. Figure 2: PRE-NMR structural ensembles and interfacial contacts of DMPC bilayer bound to opposite sides of catalytic domain. ( a ) The ensemble of 14 structures of MMP-12 positioned with its β-face on the bilayer was selected from the MD trajectory of Supplementary Movie 1 . Backbone segments that contact the bicelles are coloured dark red. The view is illustrated as a stereo pair in Supplementary Fig. 9a . ( b ) The ensemble of 14 structures of MMP-12 bound with its α-face engaging the bilayer with green segments of the S 1 ′ and V–B loops was selected from the MD trajectory of Supplementary Movie 2 . This view is illustrated as a stereo pair in Supplementary Fig. 9b . ( c ) A structure from a (viewed along the arrow in a ) is marked with interfacial contacts which are populated in at least 64% of the final structures. Hydrophobic contacts are plotted with dot surfaces. Hydrogen bonds and salt bridges are plotted with broken lines. Nitrogen, phosphorous and oxygen atoms are coloured blue, gold and red, respectively. See Supplementary Fig. 2 for a three-dimensional (3D), rotatable view. ( d ) A structure from b in the α orientation is marked with interfacial contacts reproduced in at least 64% of the final structures. See Supplementary Fig. 3 for a 3D, rotatable view. Full size image Table 1 Structural statistics of PRE-based structural ensembles. Full size table The breadth of interfaces and shallow contacts with lipid head groups ( Table 2 ) suggest reversible association with the bilayer. The α- and β-interfaces bury 2,070 and 2,530 Å 2 of surface area, respectively, making them larger than most interfaces of phospholipid recognition domains [41] . The interacting loops of MMP-12 generally are positioned with backbone among the choline head groups ( Fig. 2a,b ) and side chains slightly deeper near the phosphodiester linkages, but not so deep as to reach the acyl chains ( Fig. 2c,d and Supplementary Figs 2 and 3 ). Reversible MMP-12 association with membranes is corroborated by the rotational correlation time ( τ c ) of bicelle-associated MMP-12 of 13.4 ns, which is only 54% larger than the 8.7 ns τ c of the free state [25] , despite the slower tumbling of the bicelles. Table 2 Interfacial contacts of phospholipid head groups with amino acids and their occupancy in the structural ensembles. Full size table The peripheral bilayer engagement by MMP-12 features hydrogen bonding, salt bridges and hydrophobic contacts with the lipid head groups ( Table 2 ). In the β-interface, Arg117 (β-strand I) and Arg127 (helix A) each form a salt bridge with a phosphate group of DMPC, while Arg165 (III–IV loop) forms salt bridges with two phosphates ( Fig. 2c , Table 2 , and Supplementary Fig. 2 ). The side chains of Arg165, Phe171 and Ile191 each form hydrophobic contacts with a choline head group, while their backbone amide groups donate hydrogen bonds to a DMPC phosphate group or ester linkage. Arg127 and Phe171 fluctuate in and out of contact with phospholipid head groups in the MD trajectories ( Supplementary Movie 1 ). The side chains of Thr154 (II–III loop) and Asn119 (I–A loop) each donate a hydrogen bond to a phosphate group and Asn119 to an ester linkage as well ( Fig. 2c , Table 2 and Supplementary Fig. 2 ). The α-interface is dominated by electrostatic interactions, displaying salt bridges between Lys177 and Lys233 and phosphate groups of DMPC molecules ( Fig. 2d , Table 2 , and Supplementary Fig. 3 ). The Lys241 side chain donates hydrogen bonds to three ester linkages, and His206 to one ester linkage. The side chain and amide of Ser207 both donate hydrogen bonds to the same phosphate group. In contrast, the side chain and amide groups of Tyr242 donate hydrogen bonds to different DMPC phosphates. The side chain amide of Asn246 donates hydrogen bonds to two DMPC phosphate groups ( Fig. 2d , Table 2 , and Supplementary Fig. 3 ). Thus, the α- and β-interfaces differ in hydrophobicity and polarity. Both sides of MMP-12 bind vesicles We tested whether both modes of MMP-12 binding of bicelles ( Figs 1 and 2 ) occur with vesicles. Membrane insertion was detected using the polarity-sensitive fluor IANBD, which increases dramatically in fluorescence emission when inserted [33] . The IANBD reporter was conjugated to single cysteine residues, designated here as site-directed fluor labelling (SDFL), with labelling yields of 94 to 100% ( Supplementary Table 1 ). Excellent NMR spectra imply native-like structure with minimal perturbation by either representative cysteine substitutions or the fluor labelling ( Supplementary Fig. 4 ), in agreement with surface mutations preserving MMP-12 intact [22] , [24] , [26] . As a negative control, IANBD was conjugated to Q139C away from both bicelle-binding sites, resulting in no significant increase of fluorescence ( Fig. 3a,b ). Greater than twofold increases ( P <0.05 by one-tailed Student’s t -test) in fluorescence ( F DMPC / F 0 ) were induced by DMPC vesicles interacting with IANBD attached to any of the four bilayer-binding loops in the β-interface, namely at N119C, G155C, A173C or G190C ( Fig. 3a,c ). The Met156 and Phe171 side chains insert among the choline head groups ( Figs 2c and 3c and Supplementary Fig. 2 ) and their alanine substitutions reduced the fluorescence to 0.57- and 0.78-fold the levels of the wild-type sequence ( P <0.05, by Student’s t -test), respectively, as reported by the fluor linked to G155C ( Fig. 3a ). Thus, the four loops around the β-sheet and hydrophobic residues therein do engage membranes. 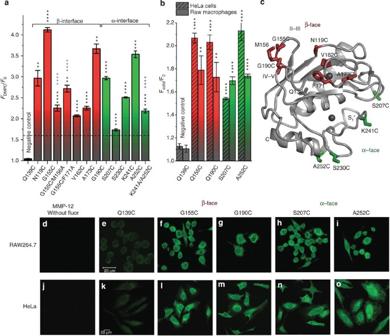Figure 3: Both α and β-interfaces of MMP-12 bind vesicles and cells. (a) Addition of DMPC vesicles (SUVs, 400 μM in monomers) increased the fluorescence of MMP-12 forms (5 nM) labelled with IANBD at the single cysteine mutations indicated. The resulting fluorescence emission,FDMPC,is plotted relative to no addition of SUVs,F0. The error bars mark the s.d. of the mean among quadruplicate samples. Differences from the Q139C control represent **P<0.005, ***P<0.0005 and ****P<0.00005 from two-tailed Student’st-testing. Blue asterisks (****) markPvalues for differences with and without the alanine mutation. The dashed line indicates significant proximity to a liposome according to elevatedF/F0ratios, judged by previous IANBD probing of the membrane-binding face of a peripheral membrane protein33. Results with bicelles are shown inSupplementary Fig. 5. (b) Addition of murine RAW 264.7 macrophages or human HeLa cells (5 million cells per well; quadruplicate samples) increased the fluorescence of MMP-12 variants labelled with IANBD where indicated. Labelling at Q139C outside the α- and β-interfaces serves as a negative control. (c) The exposed residues that were mutated and conjugated to the fluorochrome in the β- and α-sites are coloured dark red and green, respectively. The negative control site, Q139C, and zinc ions are coloured grey. (d,j) Confocal fluorescence images for cells (located by differential interference contrast) with no added protein are shown. (e–i) RAW 264.7 macrophages were incubated with IANBD-conjugated MMP-12 single cysteine variants and imaged by confocal microscopy. The scale bars represent 20 μm. (k–o) HeLa cells were incubated with the labelled MMP-12 variants and imaged. Figure 3: Both α and β-interfaces of MMP-12 bind vesicles and cells. ( a ) Addition of DMPC vesicles (SUVs, 400 μM in monomers) increased the fluorescence of MMP-12 forms (5 nM) labelled with IANBD at the single cysteine mutations indicated. The resulting fluorescence emission, F DMPC, is plotted relative to no addition of SUVs, F 0 . The error bars mark the s.d. of the mean among quadruplicate samples. Differences from the Q139C control represent ** P <0.005, *** P <0.0005 and **** P <0.00005 from two-tailed Student’s t -testing. Blue asterisks (****) mark P values for differences with and without the alanine mutation. The dashed line indicates significant proximity to a liposome according to elevated F/F 0 ratios, judged by previous IANBD probing of the membrane-binding face of a peripheral membrane protein [33] . Results with bicelles are shown in Supplementary Fig. 5 . ( b ) Addition of murine RAW 264.7 macrophages or human HeLa cells (5 million cells per well; quadruplicate samples) increased the fluorescence of MMP-12 variants labelled with IANBD where indicated. Labelling at Q139C outside the α- and β-interfaces serves as a negative control. ( c ) The exposed residues that were mutated and conjugated to the fluorochrome in the β- and α-sites are coloured dark red and green, respectively. The negative control site, Q139C, and zinc ions are coloured grey. ( d , j ) Confocal fluorescence images for cells (located by differential interference contrast) with no added protein are shown. ( e – i ) RAW 264.7 macrophages were incubated with IANBD-conjugated MMP-12 single cysteine variants and imaged by confocal microscopy. The scale bars represent 20 μm. ( k – o ) HeLa cells were incubated with the labelled MMP-12 variants and imaged. Full size image To validate the α-interface, IANBD was conjugated to a position in the V–B loop or to one of the three residues after helix B in the long S 1 ′ loop. The fluor at each site underwent large fluorescence increase on addition of DMPC liposomes. Significant enhancements of at least 2.8, 1.6, 2.5 or 3.3-fold with P <0.05 by one-tailed Student’s t -test were observed for labelling at S207C, S230C, K241C or A252C, respectively ( Fig. 3a ). This suggests that the IANBD group at each of these four sites inserted directly into vesicular membranes. However, the insertion was shallower for the S230C label, suggesting greater distance from the vesicle. The Ala substitution of Lys241 decreased the fluorescence to 0.81-fold ( Fig. 3a , P <0.05 by Student’s t -test), consistent with hydrogen bonding and charge complementarity with phospholipid head groups ( Fig. 2d ). Together this confirms that the S 1 ′ and V–B loops of the α-face bind lipid bilayers. MMP-12 binds cells by the α- and β-faces We investigated whether MMP-12 binds cells by the α and β-interfaces using a cell-based SDFL approach [34] . We compared HeLa cells with RAW 264.7 macrophages that secrete MMP-12. The IANBD probe emits dramatically brighter fluorescence in hydrophobic compartments, vesicles and cells [33] , [34] , [42] , but did not insert itself into plasma membranes when free ( Supplementary Fig. 6 ) and only minimally, if at all, when linked to MMP-12(Q139C) ( Figs 3b,e,k and 4 ). This implies that IANBD does not promote cell membrane binding. The two most bilayer-responsive sites were tagged with IANBD in each of the two membrane interfaces: G155C or G190C in the β-interface or S207C or A252C in the α-interface ( Fig. 3c ). Addition of either cell type markedly brightened the cellular fluorescence emission of the fluor-conjugated MMP-12, in contrast to the Q139C-labelled negative control ( Fig. 3b ). This strongly suggests that the catalytic domain of MMP-12 binds the cells and that this occurs via both the membrane-binding α- and β-interfaces. 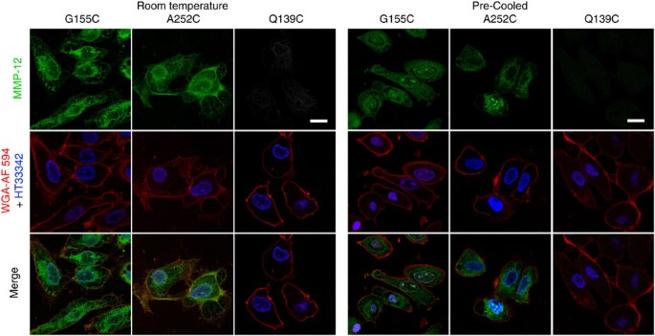Figure 4: MMP-12 binds plasma membranes, is internalized to hydrophobic compartments including the nuclear envelope and enters the nucleus. The cellular distribution of MMP-12 was visible by confocal microscopy using the enzyme labelled with IANBD on its β-face at G155C or α-face at A252C, but not when labelled outside the membrane-binding surfaces at Q139C. HeLa cells were labelled to colour the outside of plasma membranes red with wheat germ agglutinin-Alexa Fluor 594 (WGA-AF 594) and the nuclei blue with Hoechst 33342 (HT33342) using Image-IT live cell labelling kit. The images shown were taken 15 min after applying MMP-12 to cells at room temperature (left images) or to cells precooled on ice for 20 min to slow down endocytosis (right images). In the images of the precooled samples, the brightness of the green channel was increased uniformly to see the much weaker green signal and internalization. Scale bars, 20 μm. Figure 4: MMP-12 binds plasma membranes, is internalized to hydrophobic compartments including the nuclear envelope and enters the nucleus. The cellular distribution of MMP-12 was visible by confocal microscopy using the enzyme labelled with IANBD on its β-face at G155C or α-face at A252C, but not when labelled outside the membrane-binding surfaces at Q139C. HeLa cells were labelled to colour the outside of plasma membranes red with wheat germ agglutinin-Alexa Fluor 594 (WGA-AF 594) and the nuclei blue with Hoechst 33342 (HT33342) using Image-IT live cell labelling kit. The images shown were taken 15 min after applying MMP-12 to cells at room temperature (left images) or to cells precooled on ice for 20 min to slow down endocytosis (right images). In the images of the precooled samples, the brightness of the green channel was increased uniformly to see the much weaker green signal and internalization. Scale bars, 20 μm. Full size image Confocal images of RAW 264.7 macrophages and HeLa cells were acquired after 2 h of incubation at 4 °C with MMP-12 conjugated to IANBD at the β or α-surface. The addition of MMP-12 labelled at G155C, G190C, S207C or A252C shows much brighter fluorescence than Q139C-labelled outside the interfaces ( Fig. 3e–i,k–o ). The fluorescence is distributed broadly throughout both cell types ( Fig. 3f–i,l–o ). The dramatic brightening of IANBD label at the α- and β-faces, but not at the remote Q139C control site, implicates membrane bilayer binding by MMP-12 in its cellular distribution. Rapid internalization of membrane-binding MMP-12 We investigated where MMP-12 is localized in HeLa cells with the aid of markers of the plasma membrane and nucleus, namely red labelling of carbohydrates decorating the cell surface and blue Hoechst 33342 staining of the nucleus. Live cells were imaged to monitor time-dependent changes in the distribution of exogenous MMP-12 catalytic domain across intact cells. The presence of the MMP-12 catalytic domain on the cytoplasmic membrane is suggested by its ringing of cells and its co-localization with carbohydrates that decorate the extracellular surface ( Fig. 4 ). The MMP-12 tagged at the α- or β-face is distributed across cytoplasmic regions with concentration in the perinuclear compartment. The consistently bright green fluorescence emission of these constructs indicates membrane insertion of IANBD emanating from either the α- or β-face. The likelihood of this being inserted into membranes is underscored by the contrasting absence of such signal from the control of MMP-12 labelled at Q139C. The MMP-12 labelled at the α- or β-interface also appears at the nuclear envelope where the polarity-sensitive dye probably inserts in the nuclear membrane. The appearance of the protease within the nucleus might suggest its association with lipids or hydrophobic species there. Bright, punctate MMP-12 staining within the nucleus is especially evident using chilled cells ( Fig. 4 ). The internalization is rapid, with the MMP-12 tagged at G155C evident inside HeLa cells within 90 s after adding the protease exogenously ( Fig. 5 ). Major accumulation of MMP-12 on the plasma membrane, in regions around the nucleus, on the nuclear envelope and within the nucleus, was apparent within 4.5 min, based on the intense fluorescence emitted by the protease labelled on its β-face. The accumulation of MMP-12 on the cell and internal organelle surfaces continued through 12 min, as evidenced by the increased orange and green brightness, respectively ( Fig. 5 ). 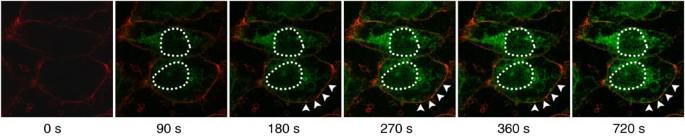Figure 5: Time-lapse confocal imaging shows IANBD-tagged MMP-12(G155C) appearing at the plasma membrane, internalized, in perinuclear regions and within the nuclei. The frames were collected through 12 min of incubation of live HeLa cells at room temperature with the labeled MMP-12 (green when associated with a membrane). The cytoplasmic membrane is stained red using WGA-AF 594. The arrowheads mark one section of plasma membrane where labelled MMP-12 appears. The dashed lines outline the cell nuclei detected by Hoechst 33342 (nuclear staining not shown). Figure 5: Time-lapse confocal imaging shows IANBD-tagged MMP-12(G155C) appearing at the plasma membrane, internalized, in perinuclear regions and within the nuclei. The frames were collected through 12 min of incubation of live HeLa cells at room temperature with the labeled MMP-12 (green when associated with a membrane). The cytoplasmic membrane is stained red using WGA-AF 594. The arrowheads mark one section of plasma membrane where labelled MMP-12 appears. The dashed lines outline the cell nuclei detected by Hoechst 33342 (nuclear staining not shown). Full size image Stable binding of active MMP-12 to the outside of the plasma membrane after repeated washing of cells is suggested by its proteolytic activity toward a linear peptide substrate ( Supplementary Fig. 7 ). This suggests that the active site remains mostly accessible while the protease is bound to the cell surface. However, several-fold lower activity of MMP-12 bound to cells is observed using a collagen V-derived substrate [43] , suggesting impaired access of the bulky, rigid substrate to the catalytic cleft. These observations are consistent with the accessibility of the central active site of the membrane-bound enzyme and the bilayer passing near the flanks of the active site ( Fig. 2 ). Effect of glycosaminoglycans on MMP-12 binding to cells The possibility of MMP-12 association with cells by binding heparan sulfate chains from proteoglycans was investigated, as these molecules are known to anchor MMP-7 (refs 18 , 19 , 44 ). When octasaccharide lengths of heparan sulfate were added up to 1.5-fold excess over 15 N-labelled MMP-12 at low ionic strength, several small chemical shift perturbations were observed. The largest of these peak shifts occur at Glu128, Tyr132 and Lys136 which form an exposed strip along helix A ( Supplementary Fig. 8a,b ). This surface corresponds to the middle of the positively charged swath on the back of MMP-7 that was hypothesized to bind heparan sulfate [44] . Since this putative GAG-binding site lies outside the bilayer interfaces ( Figs 1 , 2 , 3 ), we investigated the possibility of bilayers and GAGs jointly anchoring MMP-12 to cells. Addition of full-length heparan sulfate to 2.5 μg ml −1 preserved at least 80% of the fluorescence signature of MMP-12 binding to RAW 264.7 macrophages ( P <0.05 by one-tailed Student’s t -test) and had no effect on MMP-12 binding to HeLa cells ( Supplementary Fig. 8c,d ). The absence of heparan sulfate competition with MMP-12 binding of HeLa cells appears consistent with the rapid internalization of a large fraction of MMP-12 ( Figs 4 and 5 ), sequestering it from exposure to the exogenous heparan sulfate. The slight competition in binding macrophages suggests that heparan sulfate proteolglycans play only a limited role in anchoring MMP-12 to macrophages. With competing heparan sulfate present, the fluorescence changes ( Supplementary Fig. 8c,d ) imply that the polarity-sensitive probe attached to the α- or β-faces continues to insert into cellular membrane bilayers. The dominant means of binding is probably directly to lipid bilayers. The modes of bilayer binding by MMP-12 permit simultaneous anchoring by GAGs, but this appears to be minor in importance with macrophages and inconsequential with HeLa cells ( Supplementary Fig. 8 ). Electrostatics and unsaturation enhance vesicle binding We explored the properties that could influence membrane association. The importance of interfacial salt bridges ( Fig. 2c,d and Table 2 ) to membrane association is evident from effects of salt on vesicle binding. Physiological saline decreased the vesicle-induced F DMPC / F 0 signature of binding at both α- and β-interfaces to 0.7-fold that at 0 mM NaCl. Addition of 1 M NaCl decreased this signature of association via the α- and β-interfaces to 0.3 and 0.4-fold the levels without NaCl, respectively ( Fig. 6a ). This corroborates the structures implicating electrostatic attraction in membrane binding via both sites ( Fig. 2c,d ). It also strongly suggests that salt frees some MMP-12 to the aqueous compartment, in equilibrium with membrane-bound forms. The slightly lower sensitivity of the β-interface to high salt is consistent with its higher proportion of buried hydrophobic surface. After correcting for the charge effects of the five cations bound to MMP-12, its electrostatic potential was calculated. This indicates positive electrostatic potential across nearly all of the β-interface and much of the α-interface ( Fig. 6b,c ), consistent with predominant attraction for the phospholipid head groups. 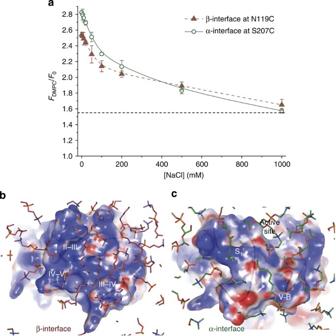Figure 6: Favourable electrostatics support MMP-12 association with vesicles. (a) Binding at both α- and β-interfaces is weakened by increasing salt concentration. MMP-12 was conjugated to the polarity-sensitive fluorophore IANBD at a single cysteine in the α- or β-interface. DMPC vesicle-induced increases of the fluorescence of the tagged variants (5 nM) withFDMPC/F0>1.55 imply the insertion of the fluorophore into the vesicles33. B-spline curves are fitted through the points. (b) The β-interface is electropositive overall. (c) Key parts of the α-interface are electropositive. The electrostatic potentials were calculated after first simulating the partial charges of the atoms surrounding the two zinc and three calcium atoms, as described in Methods. Dark blue represents +3 kT/e, while red represents −3 kT/e. The region containing DMPC head groups is shown in the foreground in the complexes. Figure 6: Favourable electrostatics support MMP-12 association with vesicles. ( a ) Binding at both α- and β-interfaces is weakened by increasing salt concentration. MMP-12 was conjugated to the polarity-sensitive fluorophore IANBD at a single cysteine in the α- or β-interface. DMPC vesicle-induced increases of the fluorescence of the tagged variants (5 nM) with F DMPC / F 0 >1.55 imply the insertion of the fluorophore into the vesicles [33] . B-spline curves are fitted through the points. ( b ) The β-interface is electropositive overall. ( c ) Key parts of the α-interface are electropositive. The electrostatic potentials were calculated after first simulating the partial charges of the atoms surrounding the two zinc and three calcium atoms, as described in Methods. Dark blue represents +3 kT/e, while red represents −3 kT/e. The region containing DMPC head groups is shown in the foreground in the complexes. Full size image The electrostatic interactions mediated by Arg117, Arg127 and Arg165 in the β-interface and Lys241 and His206 in the α-interface ( Fig. 2c,d ) were also tested by adding negatively charged lipids found in plasma membranes. The SDFL vesicle-binding assay used MMP-12 labelled with IANBD at G190C or S207C to respond to binding near the β or α-site, respectively. Additions of negatively charged lipids to 8% (w/w) consistently boosted the fluorescence evidence of insertion into DMPC or POPC vesicles by the reporter placed at either the β- or α-face ( Fig. 7 ). Cholesterol sulfate typically introduces the largest of these fluorescence increases, which are ≥1.07-fold ( P <0.05 by one-tailed Student’s t -test). The increases from addition of phosphatidyl serine are also statistically significant ( Fig. 7 ). The most significant increases of ≥1.2-fold ( P <0.05 by Student’s t -test) are from the CS and PS introduced to the DMPC vesicles and reported by IANBD in the α-interface at S207C ( Fig. 7a ). Together these results suggest that MMP-12 affinity for bilayers may be dominated by electrostatic complementarity rather than affinity for a specific lipid ligand. 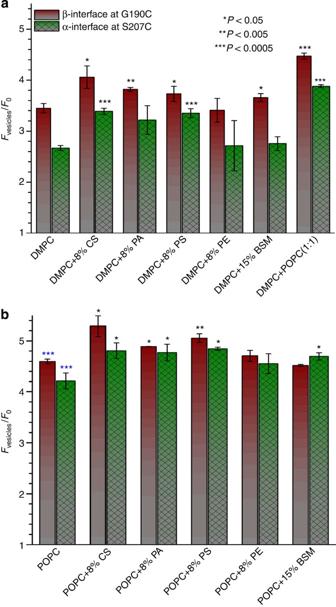Figure 7: MMP-12 association with vesicles is enhanced by unsaturated acyl chains and negatively charged lipids. (a) Vesicles of pure DMPC or mixed with another lipid were incubated with MMP-12 conjugated to IANBD at G190C (red columns) to respond to membrane binding at the β-interface or at S207C (green, cross-hatched columns) at the α-interface. The resulting fluorescence is reported relative to no addition of SUVs,F0. The negatively charged lipid additions were cholesterol sulfate (CS), phosphatidic acid (PA) or phosphatidyl serine (PS). The zwitterionic additions were phosphatidyl ethanolamine (PE), brain sphingomyelin (BSM) and POPC. The means and s.d. of triplicate measurements are shown. ThePvalues from two-tailed Student’st-testing are calculated for differences from the control without addition, that is, DMPC or POPC only, at left. (b) Binding of the tagged forms of MMP-12 to SUVs of POPC with the same lipid additions used ina. The blue asterisks refer to the differences from DMPC. Figure 7: MMP-12 association with vesicles is enhanced by unsaturated acyl chains and negatively charged lipids. ( a ) Vesicles of pure DMPC or mixed with another lipid were incubated with MMP-12 conjugated to IANBD at G190C (red columns) to respond to membrane binding at the β-interface or at S207C (green, cross-hatched columns) at the α-interface. The resulting fluorescence is reported relative to no addition of SUVs, F 0 . The negatively charged lipid additions were cholesterol sulfate (CS), phosphatidic acid (PA) or phosphatidyl serine (PS). The zwitterionic additions were phosphatidyl ethanolamine (PE), brain sphingomyelin (BSM) and POPC. The means and s.d. of triplicate measurements are shown. The P values from two-tailed Student’s t -testing are calculated for differences from the control without addition, that is, DMPC or POPC only, at left. ( b ) Binding of the tagged forms of MMP-12 to SUVs of POPC with the same lipid additions used in a . The blue asterisks refer to the differences from DMPC. Full size image Given the large areas of the interfaces, the effect of membrane fluidity on insertion was examined. Addition of zwitterionic phosphatidyl ethanolamine and brain sphingomyelin from plasma membranes preserved the levels of fluorescence from the labelled MMP-12 associated with vesicles ( Fig. 7 ). POPC, however, which contains a 9- cis double bond in its oleic acid chain at sn -2, introduced the largest enhancement of binding-induced fluorescence increase. POPC mixed 1:1 with DMPC increased F liposomes / F 0 by ≥1.25-fold with P <0.05 ( Fig. 7a by one-tailed Student’s t -test). Vesicles entirely of POPC boosted the fluorescence over DMPC vesicles by ≥1.3-fold ( Fig. 7 , P <0.05 by Student’s t -test). Either the greater membrane fluidity or the 13% larger effective area of the POPC head group [45] may allow MMP-12 better access to its shallow mode of binding or deeper insertion of the fluor among the fatty acyl chains. Thus, cell membranes containing negative charge and unsaturated lipids like POPC appear to be especially attractive to MMP-12. TIMP-2 competes with membrane bilayers for MMP-12 The resistance of MMP-7, -8 and -9 to inhibition by TIMPs when bound to cells [16] , [17] , [18] prompted us to investigate the possibility of steric conflict between the membrane association and TIMP-02 binding of MMP-12. More than 70% of the activity of MMP-12 catalytic domain on the cell surface is, however, sensitive to inhibition by TIMP-02 ( Supplementary Fig. 7 ). Both structural modes of bilayer binding by MMP-12 were superimposed on the crystal structure of MMP-13 bound to TIMP-2 (ref. 46 ). This overlay suggests that the AB loop of TIMP-2 that reaches between the IV–V and III–IV loops of MMPs would clash sterically with the bound bilayer, as these two loops are integral to the β-interface ( Fig. 8a ). The C-terminal domain of TIMP-2 reaches beyond the S 1 ′ loop of the MMP to approach the adjoining V–B loop closely to clash sterically with bilayer binding across this part of the α-interface ( Fig. 8b ). Moreover, preincubation of fluor-tagged MMP-12 variants with TIMP-2 interfered in the vesicle-induced increase of the fluorescence of IANBD placed at S207C and G190C. The bulky C-terminal domain of TIMP-2 next to the V–B loop ( Fig. 8b ) disrupted most of the fluorescence increase from bilayer penetration by the fluor linked to S207C ( Fig. 8c ), conservatively falling to 0.48-fold of the unperturbed level ( P ≤0.05 by one-tailed Student’s t -test). The next largest steric clash predicted, that is, from the AB loop of TIMP-2 adjacent to the IV–V loop of MMP-12 ( Fig. 8a ), halved the vesicle-induced fluorescence of the fluor at G190C ( Fig. 8c ), conservatively falling to 0.67-fold the level without TIMP-2 ( P ≤0.05 by Student’s t -test). Hence, the bilayer and TIMP-2 sites are structurally overlapping and functionally competitive. 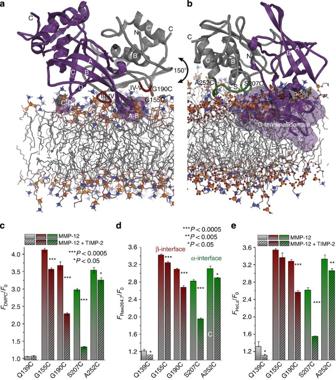Figure 8: The inhibitor TIMP-2 competes with membranes for binding beside the catalytic cleft while MMP-12 remains bound to the bilayers. (a) The structure of MMP-12 (grey) bound to the bilayer model at the β-interface (dark red loops) is superimposed on the crystal structure of the complex of TIMP-2 (purple) with MMP-13 (PDB ID 2e2d)46. The TIMP-2 surface in steric conflict is transparent purple. (b) The rotated structure of MMP-12 bound to the bilayer model at the α-interface (green loops) is superimposed on the TIMP-2-MMP-13 crystal structure. The surface of the TIMP-2 domain in steric conflict with the bilayer is transparent purple. (c) TIMP-2 competes with vesicles for binding contacts at either end of the catalytic cleft of MMP-12, while MMP-12 remains bound to the vesicles. Fluorescence increases of each MMP-12 variant (5 nM) conjugated to IANBD on incubation with DMPC SUVs are plotted, without or with preincubation with 15 nM of the tight-binding TIMP-2 inhibitor (striped bars). The means and s.d. of triplicate measurements are plotted. ThePvalues marked are from two-tailed Student’st-testing. (d) TIMP-2 complexes with MMP-12 labelled with IANBD bind RAW 264.7 macrophages robustly. Each MMP-12 variant (20 nM) was incubated 6 h with TIMP-2 (50 nM) at 23 °C before 30 min of incubation with cells on ice and detection at room temperature. The means and s.d. of quadruplicate measurements are shown. (e) TIMP-2 complexes with labelled MMP-12 (n=4) persist in binding HeLa cells as well. Figure 8: The inhibitor TIMP-2 competes with membranes for binding beside the catalytic cleft while MMP-12 remains bound to the bilayers. ( a ) The structure of MMP-12 (grey) bound to the bilayer model at the β-interface (dark red loops) is superimposed on the crystal structure of the complex of TIMP-2 (purple) with MMP-13 (PDB ID 2e2d) [46] . The TIMP-2 surface in steric conflict is transparent purple. ( b ) The rotated structure of MMP-12 bound to the bilayer model at the α-interface (green loops) is superimposed on the TIMP-2-MMP-13 crystal structure. The surface of the TIMP-2 domain in steric conflict with the bilayer is transparent purple. ( c ) TIMP-2 competes with vesicles for binding contacts at either end of the catalytic cleft of MMP-12, while MMP-12 remains bound to the vesicles. Fluorescence increases of each MMP-12 variant (5 nM) conjugated to IANBD on incubation with DMPC SUVs are plotted, without or with preincubation with 15 nM of the tight-binding TIMP-2 inhibitor (striped bars). The means and s.d. of triplicate measurements are plotted. The P values marked are from two-tailed Student’s t -testing. ( d ) TIMP-2 complexes with MMP-12 labelled with IANBD bind RAW 264.7 macrophages robustly. Each MMP-12 variant (20 nM) was incubated 6 h with TIMP-2 (50 nM) at 23 °C before 30 min of incubation with cells on ice and detection at room temperature. The means and s.d. of quadruplicate measurements are shown. ( e ) TIMP-2 complexes with labelled MMP-12 ( n =4) persist in binding HeLa cells as well. Full size image Much less competition was observed when probing membrane-binding loops that do not meet TIMP-2. The TIMP-2-induced attenuation of fluorescence of IANBD at G155C and A252C, which are outside the area of direct steric clash with TIMP-2 binding, are much smaller ( Fig. 8c ). TIMP-2 attenuates the vesicle-induced fluorescence of IANBD at G155C to 0.89-fold conservatively ( P ≤0.05 by one-tailed Student’s t -test). Thus, TIMP-2 competition with membrane binding is minimal at the G155C or A252C sites remote from the TIMP-2 binding interface, medium where there is moderate steric conflict (G190C of the IV–V loop) and large where the steric conflict is also large (S207C of the V–B loop). This suggests that MMP-12 remains bound to the vesicle, but rotates on the membrane to accommodate the TIMP-2 obstacle spanning the active site. TIMP-2 competition with MMP-12 binding to cells was examined. The patterns of cell-induced fluorescence of the IANBD-labelled MMP-12 variants, without and with preincubation with TIMP-2 ( Fig. 8d,e ), are similar to the patterns of vesicle-induced fluorescence. After preincubation of TIMP-2 with MMP-12, the high and continuing cell-induced fluorescence of the labels at G155C, G190C and A252C ( Fig. 8d,e ) implies that TIMP-2-inhibited MMP-12 continues to bind macrophages and HeLa cells. The fluorescence response of the label at G190C or S207C to cells appears to be less sensitive to TIMP-2 than the response to vesicles ( Fig. 8c–e ). For example, TIMP-2 bound to MMP-12 attenuates the fluorescence of IANBD at G190C induced by RAW 264.7 macrophages only to 0.88-fold ( P <0.05 by one-tailed Student’s t -test) and of IANBD at S207C only to 0.72-fold ( P <0.05 by Student’s t -test). This suggests the persistence of cell binding by MMP-12 despite steric competition from TIMP-2, and further suggests compensatory adjustments of MMP-12 binding to cellular membranes, such as rotations to decrease steric conflict with the TIMP-2 bound. MMP-12 has been observed to bind diverse membrane bilayers consistently via two opposing surfaces of its catalytic domain, that is, using bicelles, vesicles, plasma membranes and nuclear membranes of cells. The modes of binding are well defined by NMR and fluorescence spectroscopic methods, revealing orientations that leave the active site open enough for peptide substrates to enter ( Figs 2 and 3 and Supplementary Fig. 1 ) and that overlap at the α-face with binding of a hydrophobic, non-competitive inhibitor [47] . This offers an unprecedented basis to account for the pericellular activity of MMP-12 around activated pulmonary macrophages [14] and HeLa cells ( Supplementary Fig. 7 ). Binding of MMP-12 directly to the plasma membranes of macrophages ( Fig. 3b,f–i,l–o ) provides a mechanism for positioning MMP-12 for juxtamembrane proteolytic release of TNF-α to stimulate inflammation in smokers’ lungs [15] . MMP-12 attachment to cellular bilayers ranging from plasma membranes, perinuclear networks and the nuclear membrane ( Fig. 4 ), as well as the time course of its appearance at these compartments ( Fig. 5 ), suggest a trafficking pathway. The progression of the trafficking in minutes and its slowing and reduction on cooling are consistent with a hypothesis of endocytosis of MMP-12 bound to membranes ( Fig. 4 ). This could account for the presence of MMP-12 in phagolysozomes of macrophages where its C-terminal domain kills ingested bacteria [1] . IANBD-tagged MMP-12 accumulates in hydrophobic, presumably membranous, regions near the nucleus, according to the brightness of the fluorescence. The inward transit of MMP-12 catalytic domain to this network and the nuclear envelope is rapid and could involve lipid-dependent trafficking pathways that help deliver MMP-12 towards the nucleus. The bright punctate staining of a few particles in the nucleus by MMP-12 labelled with IANBD in either of its membrane interfaces ( Fig. 4 ) corroborates the report of MMP-12 entry into the nucleus to act as a transcription factor [2] . These particles, whether containing chromatin or otherwise, must have hydrophobic surfaces into which the polarity-sensitive fluor on MMP-12 inserts. Indeed, the nucleus contains diverse lipids [48] . The intracellular transit of MMP-12 in HeLa cells and macrophages ( Figs 3 and 4 ) suggests that the trafficking might occur in cases of inflammation beyond the antiviral response [2] . Numerous reports of MMP-1, -2, -3, -9, -13, -14 and -26 in nuclei [27] , as well as putative nuclear localization signals noted in MMP-1, -2, -3, -8, -10, -13, -14, -16, -17, -19, -20, -23 and -24 (ref. 49 ) suggest nuclear localization by more MMPs. The electrostatic attraction of MMP-12 for bilayers is analogous to well-characterized peripheral membrane proteins. Cytochrome c shuttles between redox partners embedded in the membrane and alternates between planar diffusion on the membrane and three-dimensional diffusion in the nearby solution where it is concentrated [50] , similar to intracellular lipid binding proteins [41] . MMP-12 may behave similarly, although with opportunity for the 137° flipping between the α and β orientations when it detaches and rebinds. While detached, MMP-12 is freed to hydrolyse its many soluble substrates being identified [2] , [3] . For perspective on surface mobility, the Rheb GTPase rotates freely about its deeply inserted farnesyl tether between modes of bilayer binding [51] . The two shallow modes of MMP-12 binding may increase its local concentration and residence time on membranes to increase the chance of encountering nearby partners and protein substrates. The shallow insertion of MMP-12 among the head groups ( Fig. 2 ) should reduce its frictional drag for faster translational diffusion across the membrane [52] . This could hasten collisions of MMP-12 with substrates or potential partners on membrane surfaces. This pattern is consistent with the halo of MMP-12 activity observed around activated macrophages [14] . The membrane-binding mechanisms described herein could be relevant to some other MMPs. For example, MMP-7 binds vesicles [21] , and MODA predicts that some loops of MMP-7 and -9 corresponding to the β-face of MMP-12 should bind membranes. The affinity of MMP-7 for bilayers [21] potentially enhances its association with uterine epithelial and cancer cells [18] , [19] , [20] . Direct binding of bilayers might also aid MMP-8 and -9 interactions with neutrophils [16] , [17] . If so, an MMP-12-like mode of binding membranes could explain why cell-bound MMP-7, -8 and -9 retain proteolytic activity yet modestly resist TIMP inhibition [17] , [18] . This hypothesis assumes that the catalytic cleft of these MMPs is also accessible to small substrates without obstruction by the bilayer ( Fig. 2 and Supplementary Figs 1b and 7 ), which is consistent with the activity of MMP-7, -8 and -9 bound to cells [16] , [17] , [19] . Binding of MMP-7, -8 or -9 to plasma membranes with sufficient affinity might sterically hinder binding of TIMP to the ends of the catalytic cleft ( Fig. 8a ). The fluorescence evidence ( Fig. 8c–e ) suggests that TIMP-inhibited MMP-12 adjusts its modes of binding to vesicles and cell membranes to avoid the steric clashes depicted in Fig. 8a,b . In summary, the MMP-12 catalytic domain binds to plasma and intracellular membranes, using two complementary structural orientations found on opposite sides of the catalytic cleft. This alternative positioning can promote its almost continuous localization near membranes and invites further studies of MMP trafficking and compartmentalized activities, for example, during inflammatory processes. The broad membrane-binding interfaces of MMP-12 are defined by favourable electrostatic and hydrophobic contacts with phospholipid head groups. The dual positioning of MMP-12 on membranes could be strategically important for activities near the membranes including pericellular shedding of TNF-α to promote inflammation [15] and entering and trafficking through cells to reach the nucleus to activate transcription [2] . Preparations of enzyme and lipid assemblies The inactivated catalytic domain of MMP-12(E219A) was expressed in E. coli without prodomain from Phe100 to Gly263 and with 15 N and 13 C labelling of NMR samples [23] . The catalytic domain was purified with cation exchange chromatography [53] on S-sepharose and folded with decreasing steps of urea while withholding 0.1 mM ZnCl 2 until the final dialysis [54] . To prepare SUVs of DMPC (Avanti Polar Lipids) at 100 mM, the DMPC was dissolved with vortexing at 42 °C, homogenized with around seven cycles of freezing and thawing, pelleted, redissolved, sonicated three times for 15 min in a bath sonicator to reach a transparent blue appearance and centrifuged to remove large unilamellar and multilamellar vesicles [55] . Bicelles were prepared by dissolving large unilamellar vesicles of DMPC with DHPC [32] with three cycles of incubation at 42 °C, followed by freezing in liquid nitrogen. NMR paramagnetic relaxation enhancements in bicelles NMR samples of 0.5 mM 15 N/ 13 C-labelled MMP-12 bearing an E219A point mutation to stabilize the protease were studied at 300 K in 20 mM imidazole (pH 6.6), 10 mM CaCl 2 and 20 μM ZnCl 2 . The NMR peak assignments used in measuring PREs were those of BioMagResBank entry 7,089 (ref. 56 ). Bicelles (1 DMPC: 2 DHPC; q =0.5; non-orienting) were used at a total phospholipid concentration of 80 mM and exhibited hydrodynamic radius of 4.8 nm (with 110 μM MMP-12 present) by dynamic light scattering using a DynaPro MSTC. The implied molecular weight of 144 kDa suggests approximately 86 DMPC molecules per bicelle and a bicelle concentration of approximately 310 μM. PRE experiments introduced 5-doxyl PC or 14-doxyl PC (Avanti Polar Lipids) to 620 μM, which is about 1.0 molecule per leaflet of the bicelle. Apparent 1 H R 2 relaxation rate constants were measured with and without doping with the spin-labelled phospholipid to estimate the PRE as Γ 2 = R 2,paramag − R 2,diamag . The relaxation rate constants were measured using a CPMG sequence that suppresses 1 H– 1 H J-couplings [57] . Two-point fitting [58] of TROSY-detected, amide proton relaxation used relaxation periods of 0 and 8 ms. HMQC detection of methyl relaxation used CPMG periods of 0, 4, 8, 12 and 16 ms. Distance restraints were obtained from the PREs (Γ 2 ) using an equation of ref. 59 simplified by ω H τ c >>1 to the form: where K is 1.23 × 10 −44 m 6 s −2 . The rotational correlation time τ c of protein–bicelle complexes was obtained from amide cross-correlation rates η xy [60] interpreted by the TRACT approach [61] . NMR-restrained rigid-body docking with DMPC bilayer The PRE-derived depth restraints were divided into separate sets at the α- and β-interfaces for separate structural calculations. The NMR structure of MMP-12(E219A) (PDB code 2POJ) [23] was used in rigid-body docking using either set of restraints. The coordinates of the bilayer with 128 DMPC molecules were those of Wohlert and Edholm [40] . A topology file for the bilayer was prepared with DMPC molecules linked by dummy atoms to permit fast torsion angle dynamics in HADDOCK [62] . PREs introduced by the doxyl PC added to bicelles were represented by distance restraints to atoms at a similar depth as the doxyl group in the acyl chains of eight DMPC molecules nearest the MMP-12. These were C1D and C2D atoms for 5-doxyl PC and C1M and C2M atoms for 14-doxyl spin labelling. Implementing rigid-body docking using HADDOCK 2.1 (ref. 63 ) required raising the limit on lipid molecules to 150 using MAXTREE. MD refinement of PRE-docked complexes The HADDOCK results provided starting structures for MD simulations using GROMACS 4.5.05 (ref. 64 ). The OPLS force field was used with the Berger lipid parameters [65] . The DMPC bilayer coordinates with 128 DMPC molecules [40] were downloaded from the Automated Force Field Topology Builder [66] , which was also used to generate the topology file for the DMPC bilayer. The complexes at the α- and β-interfaces were solvated with 9,619 or 9,256 TIP3P water molecules, respectively. The solvated systems were energy minimized, eight Cl − counter ions added to neutralize the charge of MMP-12, and minimized again. The first 200 ps of equilibration used the NVT ensemble and maintained 298 K by velocity scaling (the Berendsen thermostat) with a temperature coupling constant (tau_t) of 0.1 ps and coupling of each group to the temperature bath. The next 1 ns of equilibration used the NPT ensemble. During the equilibration period of 200 ps of the NVT ensemble and 1 ns of the NPT ensemble, positional restraints (spring constant of K pr =1,000 kJ mol −1 nm −2 ) were maintained on the backbone of MMP-12. The linear constraint solver method constrained all bond lengths, with a 2 fs integration step. The 15 ns production phases of the simulations avoided positional restraints and used the NPT ensemble. Pressure regulation to 1.0 bar in each direction used semi-isotropic coupling and a pressure coupling constant (tau_p) of 5.0 ps. The loose dihedral restraints used in determining the NMR structure of MMP-12 (ref. 23 ) and distance restraints to Zn 2+ and Ca 2+ ( Table 1 ) were applied during the 15 ns production phase of the trajectories. Analyses were performed using GROMACS tools. Fourteen snapshots in best agreement with the PRE-derived distance restraints were drawn from 2 ns segments of the trajectories to represent the experimentally most probable ensembles. Site-directed fluorchrome labelling Single cysteine mutations were prepared with the QuikChange approach and using PCR master mix (Stratagene). Addition of 2-mercaptoethanol to the folding protocol [54] boosted the yield. The single cysteine variants of MMP-12(E219A) at 1 μM (in fluorescence buffer of 20 mM Tris, pH 7.2, 5 mM CaCl 2 , 0.1 mM ZnCl 2 ) were conjugated at 4 °C overnight with 10 μM IANBD (Invitrogen) [33] according to the manufacturer’s protocol with excess 2-mercaptoethanol in the dark in an anaerobic chamber under vacuum. The derivatization of each cysteine variant proceeded to 94 to 100% completion ( Supplementary Table 1 ). The unreacted IANBD was readily removed by desalting on Sephadex G-25 (Sigma) [67] . Fluorescence changes detected by plate reader Fluorescence assays of interactions used quadruplicate samples of 5 nM of IANBD-labelled MMP-12 at 25 °C in 20 mM Tris, pH 7.2, 5 mM CaCl 2 and 0.1 mM ZnCl 2 . Excitation and detection wavelengths were 478 and 541 nm, respectively [33] , monitored with a BioTek Synergy MX plate reader. Assays using liposomes added them to 400 μM concentrations of lipid monomers. Assays using bicelles (1 DMPC:2 DHPC) at 55 mM total phospholipid were estimated to be around 100 μM in bicelles using the revised bicelle model of Glover et al. [30] Excess TIMP-2 (Syd Labs, Boston) was added using several hours of preincubation with MMP-12 variants in order for the slow binding to equilibrate. For plate-based assays of cell-increased fluorescence of IANBD-labelled MMP-12(E219A), approximately 5 million mammalian cells were added per well. 20 nM MMP-12 variant was preincubated 6 h with 50 nM TIMP-2 at 23 °C before incubating 30 min with the cells on ice and detecting fluorescence at room temperature. The data points plotted in the bar charts are means±s.d. of triplicate or quadruplicate measurements. The process of statistically comparing the significance of differences in membrane or cell-increased fluorescence of IANBD-labelled MMP-12 first applied F-testing for equal or unequal variances. Then the data were analysed by Student’s t -test with equal or unequal variance accordingly, using Microsoft Excel. The significance of differences in measurements was evaluated using two-tailed Student’s t -tests. One-tailed Student’s t -tests established the size of significant changes in fluorescence due to the treatment. Culture of RAW 264.7 and HeLa cell lines The mouse monocyte/macrophage cell line RAW 264.7 and the human HeLa cervical adenocarcinoma cell line were obtained from the American Type Culture Collection (Manassas, VA) and were free of mycoplasma. Cells were maintained in Dulbecco’s modified Eagle’s high glucose medium (DMEM, Life Technologies, Grand Island, NY) supplemented with 10% (v/v) fetal bovine serum (Sigma) and 50 μg ml −1 gentamicin (APP Pharmaceuticals, Schaumburg, IL)) and cultured at 37 °C in a humidified atmosphere with 5% CO 2 . Cells were harvested with TrypLE (Life Technologies) and DMEM media was added to the suspension. Cells were resuspended in 20 mM Tris pH 7.2, 5 mM CaCl 2 , 0.1 mM ZnCl 2 following centrifugation, counted and adjusted to the appropriate concentration. Fluorescent imaging of MMP-12 association with cells Cells to be fixed were grown overnight to 80% confluency on sterile glass cover slips. The cells were placed on ice to impede membrane trafficking. After washing three times with ice-cold DMEM without phenol red, the cells were incubated with staining agents. For the images of Fig. 3 , cultures of RAW 264.7 macrophages and HeLa cells were incubated on ice with 100 nM MMP-12 variants in DMEM without phenol red for 2 h, followed by washing five times with PBS on ice, fixing for 10 min with 4% paraformaldehyde and imaging with a Zeiss LSM 510 Meta confocal microscope. To examine the time course of MMP-12 internalization in living cells, HeLa cells were grown overnight to 60–80% confluency on sterile MatTek (Ashland, MA) glass-bottom culture dishes. These cells were washed three times with DMEM without phenol red and incubated 10 min (at 37 °C, 5% CO 2 ) with the Image-It kit (Life Technologies) comprising the Alexa Fluor 594 conjugate of wheat germ agglutinin (WGA-AF 594) at 5 μg ml −1 to label the outer face of the plasma membranes red and 2 μM of Hoechst 33342 to label double-stranded DNA and nuclei blue. The cells were then washed three times with 20 mM Tris, pH 7.2, 5 mM CaCl 2 and 0.1 mM ZnCl. A culture dish was then placed on the stage of a Leica TCP SP8 MP inverted spectral confocal microscope equipped with 405 nm and tunable white light lasers. The excitation/emission band-pass wavelengths used to detect Hoechst 33342, IANBD and Alexa Fluor 594 WGA were set to 405/415–470, 472/485–525 and 594/610–680 nm, respectively. After taking the first multichannel image (time point 0), 100 nM of the IANBD-labelled MMP-12 variant was added and images collected at 21–22 °C every 90 s over a period of ~20 min using the settings mentioned above. To slow down MMP-12 trafficking, cultured HeLa cells were placed on ice for 20 min and then subjected to the same staining and time-lapse imaging protocols. Electrostatic calculations The MMP-12 crystal structure (PDB code 1JK3) [37] was used for calculating partial charges on atoms surrounding the two zinc ions and three calcium ions. At the active site, the inhibitor was removed from 1JK3 and two bound waters introduced where two the oxygen ligands from the inhibitor had been. The charges and radii at the two zinc and three calcium binding sites were parameterized by combined application of Ambertools module MCPB/MTKPP [68] and Gaussian 09 (Revision B.01) at the B3LYP/6-31G* level. The partial charges surrounding these five cations were transferred to the coordinates (PQR files) of the α- and β-complexes of MMP-12 with bilayer models. Elsewhere, the Amber f99SB [69] radii and charges were applied to the assemblies. Electrostatic potentials were calculated using the Adaptive Poisson-Boltzmann Solver [70] at 298 K and ionic strength of 30 mM. The protein and solvent dielectric constants were set to 2.0 and 78.54, respectively. The protonation state was set to pH 7. Accession codes : The experimental restraints and structural ensembles of the MMP-12 complexes with DMPC bilayer have been deposited in the Protein Data Bank under accession numbers 2MLR and 2MLS for the α and β-interfaces, respectively. How to cite this article: Koppisetti, R. K. et al. Ambidextrous binding of cell and membrane bilayers by soluble matrix metalloproteinase-12. Nat. Commun. 5:5552 doi: 10.1038/ncomms6552 (2014).